Photonic spin Hall effect in hyperbolic metamaterials for polarization-controlled routing of subwavelength modes The routing of light in a deep subwavelength regime enables a variety of important applications in photonics, quantum information technologies, imaging and biosensing. Here we describe and experimentally demonstrate the selective excitation of spatially confined, subwavelength electromagnetic modes in anisotropic metamaterials with hyperbolic dispersion. A localized, circularly polarized emitter placed at the boundary of a hyperbolic metamaterial is shown to excite extraordinary waves propagating in a prescribed direction controlled by the polarization handedness. Thus, a metamaterial slab acts as an extremely broadband, nearly ideal polarization beam splitter for circularly polarized light. We perform a proof of concept experiment with a uniaxial hyperbolic metamaterial at radio-frequencies revealing the directional routing effect and strong subwavelength λ /300 confinement. The proposed concept of metamaterial-based subwavelength interconnection and polarization-controlled signal routing is based on the photonic spin Hall effect and may serve as an ultimate platform for either conventional or quantum electromagnetic signal processing. Designing a material environment at the nanoscale allows one to achieve precise control over propagation of electromagnetic waves by tuning their amplitudes and phases when the electromagnetic field interacts with nanostructures [1] , [2] . The approach based on discrete nanoresonators and their arrangements in various kinds of metamaterials has already resulted in many applications, such as cloaking [3] and perfect lensing [4] , as well as spontaneous emission and nonlinearity engineering [5] . The direction of light propagation can also be controlled by the polarization degree of freedom [6] , [7] , [8] , [9] , [10] , [11] , [12] . In particular, when circularly polarized light interacts with specifically designed nanostructured metasurfaces that break spatial inversion symmetry, photons of different polarizations (optical spin) may take different trajectories, in close analogy to the spin Hall effect for electrons [7] , [8] , [9] , [10] , [11] . In terms of manipulation of emission properties, anisotropic metamaterials with hyperbolic isofrequency surfaces have been proposed for nonresonant enhancement of the spontaneous emission rate [13] , which are fundamentally limited only by the basic dimensionality of an artificial unit cell [14] and nonlocal effects [15] . Such anisotropic metamaterials have different signs of the longitudinal ( ε ‖ ) and transverse ( ε ⊥ ) components of the effective permittivity tensor and have been realized as nanowire arrays [16] or layered metal–dielectric structures [13] ( Fig. 1 ). Hyperbolic metamaterials have been demonstrated for sub-diffraction imaging (hyper-lensing) [17] , directional single photon emission [18] , subwavelength interference pattern formation [19] and enhancement of nonlinear optical effects [20] . 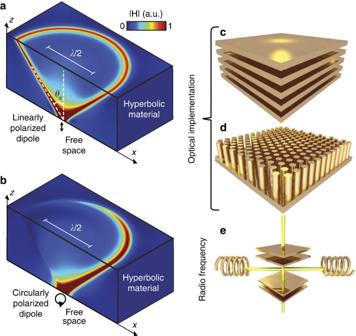Figure 1: Basic concepts. (a,b) Intensity distribution of the dipole radiating in the vicinity (atλ/50 distance from the interface) of a slab of a metamaterial with hyperbolic dispersion (ε‖=εx,y=−1,ε⊥=εz=1) in the case of (a) linear and (b) circular polarization. The simulated intensity cross-sections are plotted. (c–e) Possible realizations of hyperbolic metamaterials in the optical regime as (c) a metal–dielectric multilayer and (d) a metal nanorod composite, and in the radio-frequency regime as (e) a lumped circuit. Figure 1: Basic concepts. ( a , b ) Intensity distribution of the dipole radiating in the vicinity (at λ /50 distance from the interface) of a slab of a metamaterial with hyperbolic dispersion ( ε ‖ = ε x,y =−1, ε ⊥ = ε z =1) in the case of ( a ) linear and ( b ) circular polarization. The simulated intensity cross-sections are plotted. ( c – e ) Possible realizations of hyperbolic metamaterials in the optical regime as ( c ) a metal–dielectric multilayer and ( d ) a metal nanorod composite, and in the radio-frequency regime as ( e ) a lumped circuit. Full size image Here, we show that a circularly polarized emitter (for example, an atom, molecule or classical antenna) near an anisotropic hyperbolic metamaterial slab will unidirectionally emit into extraordinary modes of the metamaterial exhibiting high density of electromagnetic states (DOS) and strong spatial localization, with the directionality of energy propagation controlled by the circular dipole handedness. The effect has been numerically demonstrated in the optical regime for metal–dielectric multilayered hyperbolic metamaterials and in the radio-frequency (RF) regime for a hyperbolic metamaterial based on lumped circuit elements. In the experimental realization, a hyperbolic metamaterial operating at 36 MHz frequency has been shown to support the selective excitation of directional and strongly confined (up to about λ /300 full width at half maximum) modes, in complete analogy to the optical phenomena. Thus, a metamaterial slab acts as an extremely broadband polarization beam splitter for circularly polarized electromagnetic fields. In particular, 27 dB (in optical frequency range) and 10 dB (in RF range) power ratios radiated in different directions were found for left-handed and right-handed circularly polarized dipoles. The demonstrated capability of polarization-controlled subwavelength routing of electromagnetic fields efficiently and directionally in an alignment free configuration can be invaluable for large-scale system integration based on emitter–metamaterial interactions, spanning from radio to optical frequency range. Directional excitation of modes in hyperbolic metamaterials In uniaxial media, optical properties, such as reflection, absorption and transmission, can be described by a diagonal permittivity tensor with ε x = ε y ≠ ε z . For metamaterial composites, these parameters are determined by the geometry and material properties of individual components and can be extracted within the effective medium theory [21] , [22] . Generally, a uniaxial anisotropic medium supports two types of waves: ordinary and extraordinary ones. Electromagnetic waves with polarization in the plane of the layers experience the permittivity ε ‖ = ε x = ε y on interaction with the metamaterial regardless of the direction of the wave vector, if spatial dispersion is neglected. At the same time, the waves with all other polarizations are governed by the permittivity ε e ( θ ), which depends on the propagation direction: where θ is the angle between the wave vector and the crystallographic axis ( Fig. 1 ). For hyperbolic metamaterials, for which ε z / ε x <0 in a certain frequency range, ε e ( θ ) diverges at the angle tan 2 θ C = if losses are ignored. This implies that at this angle, the DOS will be infinite since it depends on ε e ( θ ), and all scattered or emitted radiation will propagate within the extraordinary mode forming a cone with an opening angle of θ C ( Fig. 1a ). In reality, material losses and nonlocal effects related to the finite thickness of the discrete constituent elements accompanying any actual realization of metamaterial, will reduce the local DOS (LDOS) of the dominating mode and broaden the angular distribution of the emission. Nevertheless, optical losses limit but not inhibit hyperbolic dispersion related effects, for example, hyperlensing [23] and the Purcell factor enhancement [13] , and can be suppressed by introduction of gain [24] , [25] . If an elliptically polarized emitter is situated in near-field proximity to the interface of the hyperbolic metamaterial ( Fig. 1 ), its emission will be efficiently coupled to the high-LDOS modes. The vectorial structure of the field of an elliptical dipole allows one to direct the emission selectively in a specific direction with appropriate choice of polarization using the near-field interference effects [9] , [26] . To simplify considerations, we restrict the discussion to a 2D emitter with a dipolar moment situated in near-field proximity of the metamaterial. Such a dipole will excite all possible plane wave modes in a metamaterial with an efficiency proportional to their LDOS and the strength of the interaction , where is the electric field of the k -th mode at the emitter location [27] . The coupling efficiency to the dominating (high LDOS) mode is given by where translational symmetry is assumed along the y axis. Thus, a destructive interference condition in the near-field can be fulfilled if p x E x + p z E z =0 and can take place for an elliptically polarized dipole coupled to the mode of the hyperbolic metamaterial having transversal and longitudinal field components. This effect is analogous to the one observed in the excitation of the modes of dielectric waveguides or surface plasmon polaritons by circularly polarized light, resulting in polarisation-controlled directionality of the waveguided modes [9] . The electric field of any transverse-magnetic guided mode close to the boundary of its waveguide satisfies , where k x and k z = i are the mode wave vectors in the x and z directions, respectively. The subwavelength width, high DOS mode in a hyperbolic metamaterial is made up of the superposition of different components with k x >> k 0 or k x <<− k 0 depending on the direction of propagation of the beam; therefore, the electric field of the guided mode at the emitter location can be approximated with , where the sign depends on the direction of propagation along the waveguide ( Fig. 2 ). It follows that, according to Equation 2, the emission from the dipole will be absent when p x / p z =− E z / E x ≈ i , which corresponds to a circularly polarized dipole with one or another sense of rotation. With hyperbolic metamaterials, however, not only directionality, but also a guiding channel is automatically selected due to the LDOS angular distribution. 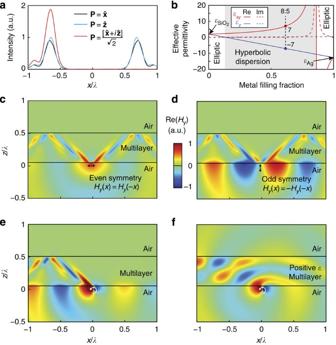Figure 2: Unidirectional signal routing in multilayer metamaterial. (a) Simulated intensity distributions on the upper boundary of the hyperbolic metamaterial slab obtained with the excitation by linear and circularly polarized dipoles. (b) The dependence of the effective permittivities of the multilayered metamaterial on the filing factor. The grey region corresponds to the spectral range of the hyperbolic dispersion (εz·εx,y<0). (c–f) Field maps of the transverse-magnetic guided mode in the metamaterial slab excited by (c) linearly polarized horizontal, (d) linearly polarized verticaland (e) circularly polarized dipolenear the hyperbolic metamaterial and (f) circularly polarized dipolenear the metamaterial with elliptic dispersion. Figure 2: Unidirectional signal routing in multilayer metamaterial. ( a ) Simulated intensity distributions on the upper boundary of the hyperbolic metamaterial slab obtained with the excitation by linear and circularly polarized dipoles. ( b ) The dependence of the effective permittivities of the multilayered metamaterial on the filing factor. The grey region corresponds to the spectral range of the hyperbolic dispersion ( ε z · ε x,y <0). ( c – f ) Field maps of the transverse-magnetic guided mode in the metamaterial slab excited by ( c ) linearly polarized horizontal , ( d ) linearly polarized vertical and ( e ) circularly polarized dipole near the hyperbolic metamaterial and ( f ) circularly polarized dipole near the metamaterial with elliptic dispersion. Full size image Hyperbolic metamaterial at optical frequencies We first consider the metamaterial realization with a metal–dielectric multilayer stack, which in the effective medium approximation constitutes a hyperbolic metamaterial with effective permittivities ε x = fε m +(1− f ) ε d and ε z =[ f / ε m +(1− f )/ ε d ] −1 , where ε m and ε d are the metal and dielectric permittivities, respectively, f is the metal filling fraction f = t m /( t m + t d ), and t m and t d are the metal and dielectric layer thicknesses, respectively. The destructive interference condition (Equation 2) can be fulfilled by a circularly polarized dipole situated near the boundary of a glass/silver multilayered structure ( =2 and ε Ag =−12.6+0.42 i at 545 nm wavelength) forming a hyperbolic metamaterial. For t m =8 nm and t d =5 nm, the hyperbolic regime is realized with ε x =7+0.08 i and ε z =−7+0.26 i ( Fig. 2b ). However, for the emitter situated in the near-field proximity of the metamaterial, an exact modelling of the structure is required because the homogeneous effective medium approximation breaks down for the description of the near-field interactions [28] , [29] . While a linearly polarized, either horizontally or vertically, emitter excites equally the extraordinary (transverse-magnetic) modes with high LDOS to the right and left from its position ( Figs 1a and 2c,d ), the circularly polarized dipole destructively interferes in one direction, depending on the polarization handedness ( Figs 1b and 2e ). This can be understood from the symmetry arguments by considering the phase relations of the fields generated by the horizontal and vertical dipoles ( Fig. 2c,d ). These fields can be intuitively summed up, and the qualitative result can be immediately inferred. The intensity clearly shows the strong directionality of the confined, subwavelength modes inside the metamaterial. The lateral confinement of the mode is about λ /15 full-width half maximum. The electromagnetic energy density distribution at the output (opposite to the emitter) interface of the metamaterial slab for different emitter polarizations clearly shows that the energy is divided equally in both directions for linearly polarized emitters, while it is radiated in a single direction when using a circularly polarized emitter ( Fig. 2a ). Changing the polarization handedness switches the direction of the emission. The contrast provided by such a polarization beam splitter is greater than 27 dB even in subwavelength dimension devices. Since the only requirement on the polarization-handedness-induced routing by the metamaterial is its hyperbolic dispersion, the reported beam splitting phenomenon is inherently broadband. To emphasize the pronounced difference between hyperbolic and elliptic dispersion regimes on the emission of a circularly polarized dipole, the same geometry of layers has been considered with different parameters in order to achieve elliptic dispersion at the given wavelength. The observed field profile shows distinctive difference compared with the hyperbolic metamaterial ( Fig. 2f ). In the elliptic regime the LDOS of extraordinary modes is similar to the LDOS of ordinary modes. While the strongly confined and directed radiation beam in the dominant extraordinary mode is excited by the circular dipole in the hyperbolic case, the elliptic metamaterial slab acts as a conventional waveguide with the directionality of the waveguided mode excitation being still observed [9] . Hyperbolic metamaterial at RF frequencies Scalability of Maxwell’s equations with respect to the operation frequencies enables the investigation of certain phenomena at much lower frequencies, where the fabrication and measurements are more straightforward. High-performance metamaterials can be constructed to achieve the required permittivity and permeability responses in the RF spectral range [30] and enable various applications, such as cloaking [31] and compact cavity resonators [32] . To understand the close analogy between current and voltage in a transmission line metamaterial and electromagnetic wave propagation in an anisotropic medium, we consider a basic unit cell of a two-dimensional transmission line metamaterial ( Fig. 3a ). 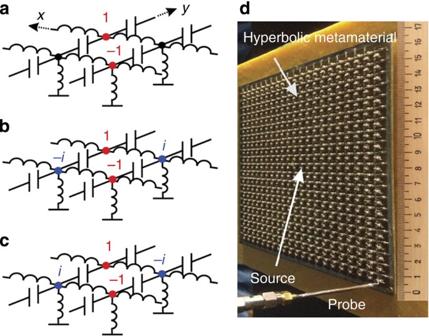Figure 3: RF metamaterial implementation. (a–c) The unit cell of the 2D transmission line metamaterial composed of lumped elements excited by (a) a linearly polarized and (b) left- and (c) right-circularly polarized dipoles. (d) Photograph of the 2D hyperbolic metamaterial prototype composed of 21 × 21 unit cells. The voltage U at one node in the grid is related to its neighbours via the Kirchhoff current law [33] : Figure 3: RF metamaterial implementation. ( a – c ) The unit cell of the 2D transmission line metamaterial composed of lumped elements excited by ( a ) a linearly polarized and ( b ) left- and ( c ) right-circularly polarized dipoles. ( d ) Photograph of the 2D hyperbolic metamaterial prototype composed of 21 × 21 unit cells. Full size image where x and y denote the node position, and Y x and Y y are the respective admittances (capacitances and inductances). The parameter Y z corresponds to the admittance of the shunt element. Equation 3 can be recast in a continuous form by replacing the discrete differences by appropriate derivatives: where S is the area of the unit cell, and is the continuous counterpart of U . Extraordinary waves of a uniaxial anisotropic medium in 2D geometry are described with a single magnetic field component =(0, H y , 0), so that the wave equation is given by where ε x ≠ ε z are the components of the medium permittivity, μ 0 is the vacuum permeability, and ω is the frequency. The complete similarity between Equation 4 and Equation 5 enables mimicking optical phenomena, emerging from Equation 5, with the RF transmission line counterpart (Equation 4). Remarkably, the hyperbolic regime in the RF metamaterial can be achieved if the chains of capacitances form the x ‘crystallographic’ axis, while the chains of inductances are in the perpendicular direction, or vice versa. The shunt admittance Y z should also have complex impedance with negligible Ohmic losses in order to achieve real effective permittivities of the array and has been chosen as an inductance in our case. The modelled magnetic field distribution in the RF hyperbolic metamaterial excited by a linearly polarized dipole ( Fig. 4a ) placed at the centre of the metamaterial shows a symmetric radiation pattern similar to the one observed in Fig. 2 , where the energy propagates equally along the direction of the extraordinary axes. Like in the optical regime, strongly directional, not symmetric magnetic field intensity distributions are excited by either left-hand or right-hand polarized dipoles ( Fig. 4b,c ). The contrast ratio of the intensity in orthogonal directions corresponds to about 10 dB, with the width of the excited mode being λ /300 (full width at half maximum). Similar behaviour was also observed in the case when the excitation antenna was outside the metamaterial ( Fig. 5a–d ). The latter configuration corresponds to the geometry considered above for optical metamaterial. 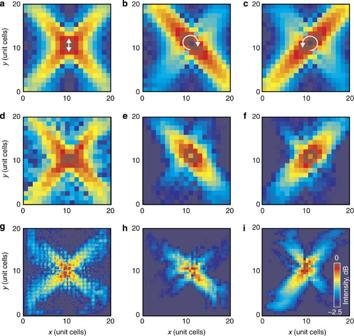Figure 4: Unidirectional signal routing in hyperbolic RF metamaterial with the emitter inside the metamaterial. The intensity distributions of the waveguided modes in the metamaterial excited by linearly polarized (left column) and circularly polarized dipoles of different handedness (middle and right columns). (a–c) Simulated intensity maps in the case of an ideal lossless metamaterial, (d–f) simulated intensity maps in the case of a metamaterial with random imperfections and (g–i) experimentally measured intensity maps. The polarization of the excitation dipoles is indicated in the figures. Figure 4: Unidirectional signal routing in hyperbolic RF metamaterial with the emitter inside the metamaterial. The intensity distributions of the waveguided modes in the metamaterial excited by linearly polarized (left column) and circularly polarized dipoles of different handedness (middle and right columns). ( a – c ) Simulated intensity maps in the case of an ideal lossless metamaterial, ( d – f ) simulated intensity maps in the case of a metamaterial with random imperfections and ( g – i ) experimentally measured intensity maps. The polarization of the excitation dipoles is indicated in the figures. 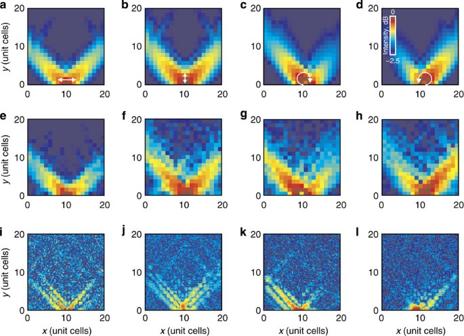Figure 5: Unidirectional signal routing in hyperbolic RF metamaterial with the emitter in the near-field of the metamaterial. The intensity distributions of the waveguided modes in the metamaterial excited by linearly polarized and circularly polarized dipoles of different handedness. (a–d) Simulated intensity maps in the case of an ideal lossless metamaterial, (e–h) simulated intensity maps in the case of a metamaterial with random imperfections and (i–l) experimentally measured intensity maps. The polarization of the excitation dipoles is indicated in the figure. Full size image Figure 5: Unidirectional signal routing in hyperbolic RF metamaterial with the emitter in the near-field of the metamaterial. The intensity distributions of the waveguided modes in the metamaterial excited by linearly polarized and circularly polarized dipoles of different handedness. ( a – d ) Simulated intensity maps in the case of an ideal lossless metamaterial, ( e – h ) simulated intensity maps in the case of a metamaterial with random imperfections and ( i – l ) experimentally measured intensity maps. The polarization of the excitation dipoles is indicated in the figure. Full size image Observation of unidirectional modes in RF metamaterial The photograph of the 2D hyperbolic metamaterial prototype composed of lumped elements and operating at the frequency f 0 =36 MHz is depicted in Fig. 3d . The effective permittivities at this frequency (see Methods) are given by L x / L z =0.33 and −1/ ω 2 L z C y =−0.33 so that this RF metamaterial operates in the hyperbolic dispersion regime. We have experimentally studied the emission of a dipole of different polarizations placed inside and in the near-field of this 2D hyperbolic metamaterial. In the ‘emitter inside’ configuration, the measured field distribution has a pronounced cross-like shape for the linearly polarized dipole ( Fig. 4g ) in agreement with the simulations. The interaction of the modes with the boundaries of the metamaterial can also be seen due to the finite size of the prototype. For the circularly polarized dipoles, the measured field exhibits unidirectional energy propagation depending on the dipole polarization handedness ( Fig. 4h,i ). The width of the excited modes in this case is similar to that excited with linearly polarized dipoles and compares well to the modelled value. In the configuration when the emitter is situated in the near-field of the metamaterial edge, the predicted behaviour for differently polarized emitters is also observed with the directionality controlled by the polarization of the dipole ( Fig. 5k,l ). To obtain better correspondence between experimental observations and the numerical model, imperfections in the realization of the metamaterial were statistically (10% distribution) included in the simulations to account for Ohmic loss in all components, fabrication imperfections and the tolerance of component nominal values. The simulated field distributions for both excitation scenarios are shown in Figs 4d–f and 5e–h . While the main trends are the same in the ideal and stochastic models, the stochastic modelling better corresponds to the experiment and confirms a slight asymmetry of the radiation patterns of right and left circularly polarized dipoles as well as enables to reproduce stronger attenuation of the guided modes due to parasitic losses in lumped elements. Metamaterials with different functionalities provide new promising solutions for a variety of applications relying on manipulation of electromagnetic fields. We have used the inherent property of hyperbolic metamaterials to support broadband, in both frequency and wave vector, electromagnetic modes [34] with high LDOS to demonstrate on-demand routing of electromagnetic signals on a deep subwavelength scale. In particular, we have shown that the new effect of near-field interference enables the broadband mapping of light in space, depending on its polarization handedness. This mapping is similar to the spin Hall effect, which has recently been considered also in optical domain for new quantum optical applications [7] , [8] , [10] , [11] employing the structured interfaces to break the inversion symmetry. In our realization, this effect is observed due to the inversion symmetry broken by the radiating dipole. The incident photons with opposite spins, determined by the handedness of the light polarization, are separated by the metamaterial in waveguided modes propagating in opposite directions, in analogy to the electron sorting by their spin in a current flow [35] . The emergence of the phenomenon was experimentally demonstrated with an RF hyperbolic metamaterial composed of lumped elements. In the optical regime, experimental realizations are possible using a subwavelength (in order to suppress higher multipoles) particle acting as a dipolar emitter, illuminated by a beam with a prescribed polarization state or appropriately designed optical nano-antenna. At lower frequencies, for example, RF range, a pair of perpendicular dipolar wire antennas, illuminated by a circularly polarized field, will act as a perfect circular dipole source. From the quantum information perspective, the emerging field of spintronics, enabling the control of individual electron spins in semiconductor structures, for example, quantum dots [36] , could serve as another excitation source for the proposed effect. The applications of the demonstrated phenomena are not limited to routing of classical optical signals. The proposed concept may be valuable for quantum information processing where large-scale quantum networks are required with efficient in/out coupling to quantum emitters of single photons [37] . Another opportunity lies in the ability of the discussed effect to detect and sort molecules by their chiral properties, which is of crucial importance for pharmacology, since molecules with the same chemical composition could have different biological activities, for example, toxicity, depending on their chirality [38] . Numerical modelling The numerical simulations of the optical metamaterials were performed using the transfer matrix approach and plane wave decomposition [39] . To model the RF hyperbolic medium, we have used the unit cell of the 2D metamaterial transmission line depicted in Fig. 3a . To mimic a hyperbolic metamaterial with effective permittivities ±0.33 at the operational frequency f 0 =50 MHz, the values of lumped elements have been chosen as C y =3.2 nF, L x =3.2 nH and L z =9.5 nH. For the grid consisting of 21 × 21 unit cells, we analytically solved the Kirchhoff equations and obtained the voltage distribution along the grid. A radiating dipole was mimicked by small current filaments, while a nearly harmonic regime of weak coupling between the dipole and the metamaterial was assumed. To mimic the linearly polarized dipole, two voltage sources with the same amplitude and opposite phases in two diagonal nodes of the structure (marked in Fig. 3a as +1 and − 1, respectively) were used. A circular dipole was implemented using four voltage sources connected to four neighbouring nodes at the centre of the array. The sources share the same amplitude but are 90° phase-shifted with respect to each other (marked in Fig. 3b,c ). The current circulation was calculated around each unit cell, which is approximately proportional to the measured magnetic field. Experimental investigations The prototype of the RF hyperbolic metamaterial composed of 21 × 21 unit cells has been fabricated using commercially available chip capacitors (RM216R71H332K C y =3.3 nF) and inductors (LQW2BHN3N3D L x =3.3 nH and LQW2BHN10NJ L z =10 nH) from Murata. The components have been mounted on a FR4 dielectric substrate ( ε r =4.4) with the help of a soldering robot Everprecision EP-SR. To provide the matching conditions at the edges, 1 Ω resistors (model ERJ6BQF1R0V from Panasonic) have been mounted. The prototype dimensions are 160 × 160 mm. For the experimental investigation, a two-port Agilent E8362C VNA has been used. One port of the VNA has been used to excite the prototype, while the second one has been used to measure the response. For the measurements with the excitation dipole outside the metamaterial, an antenna based on a current loop (8 mm diameter corresponding to λ /1,250) was brought in almost touching contact with the edge of the metamaterial. For the measurements with the excitation dipole inside the metamaterial, the electric current was directly injected into the central nodes of the structure. The experimental difference between the ‘emitter inside’ and ‘emitter in the near-field’ excitation schemes is the finite size of the loop used for the excitation in the latter case, which may be responsible for the spread of the radiation pattern (modal confinement). To achieve the dipoles with different polarizations, we have used the commercially available splitters (SBTCJ-1 W+ and JSPQ-65 W+) from Mini-Circuits. The components have been mounted on an additional circuit board (FR4, ε r =4.4) connected between the first port of the VNA and the excitation antennas. The second port of the VNA has been used to measure the signal collected by a magnetic probe at a distance of 1 mm above the top surface of the prototype using an automatic, mechanical, near-field scanner. A magnetic probe was used for the measurements; therefore, the magnetic field distribution was mapped. The field has been measured along the metamaterial surface with a 4 mm step ( λ /2,500). During the experimental measurements, we observed the simulated metamaterial behaviour at the frequency of 36 MHz instead of 50 MHz. This red shift originates from the presence of a dielectric substrate and the finite width of microstrip lines used for the interconnection of lumped elements, and usually needs to be taken into account either phenomenologically or directly from experiments [40] , [41] . The impedance of a microstrip line of width 0.8 mm implemented on an FR4 substrate of 1.5 mm thickness is 92 Ω and results in the red shift of the resonance towards 36 MHz, as was confirmed with the Sonnet@ simulations. How to cite this article: Kapitanova, P. V. et al . Photonic spin Hall effect in hyperbolic metamaterials for polarization-controlled routing of subwavelength modes. Nat. Commun. 5:3226 doi: 10.1038/ncomms4226 (2014).